PINK1 autophosphorylation upon membrane potential dissipation is essential for Parkin recruitment to damaged mitochondria Dysfunction of PINK1, a mitochondrial Ser/Thr kinase, causes familial Parkinson's disease (PD). Recent studies have revealed that PINK1 is rapidly degraded in healthy mitochondria but accumulates on the membrane potential (ΔΨm)-deficient mitochondria, where it recruits another familial PD gene product, Parkin, to ubiquitylate the damaged mitochondria. Despite extensive study, the mechanism underlying the homeostatic control of PINK1 remains unknown. Here we report that PINK1 is autophosphorylated following a decrease in ΔΨm and that most disease-relevant mutations hinder this event. Mass spectrometric and mutational analyses demonstrate that PINK1 autophosphorylation occurs at Ser228 and Ser402, residues that are structurally clustered together. Importantly, Ala mutation of these sites abolishes autophosphorylation of PINK1 and inhibits Parkin recruitment onto depolarized mitochondria, whereas Asp (phosphorylation-mimic) mutation promotes mitochondrial localization of Parkin even though autophosphorylation was still compromised. We propose that autophosphorylation of Ser228 and Ser402 in PINK1 is essential for efficient mitochondrial localization of Parkin. Parkinson's disease (PD) is one of the most pervasive neurodegenerative diseases, affecting 1% of the population over the age of 65. PD commonly arises sporadically; however, in some cases the disease is familial and inherited. PINK1 and PARKIN are causal genes for hereditary (that is, autosomal recessive) early-onset PD [1] , [2] . Studies on their functions can consequently provide important insights into the molecular mechanism of disease pathogenesis. Although the cause of sporadic PD is likely complex, numerous evidences link mitochondrial dysfunction to its pathogenesis; for example, a moderate deficit in mitochondrial electron transport chain complex activity and mutations/deletions of mitochondrial DNA in PD patients have repeatedly been reported [3] , [4] . In 2008, Narendra et al . [5] reported that Parkin translocates to and degrades depolarized mitochondria following uncoupler treatment. Although this experimental system is an artificial one, it is commonly used as a cellular experimental model for PD that might reflect the intrinsic damage in electron transport chain and the mutations/deletions in mitochondrial DNA that inevitably lead to a decrease in membrane potential (ΔΨm). Newly emergent evidence has shown that PINK1- and Parkin-dependent ubiquitylation has a pivotal role in the quality control of mitochondria, which suggests that dysfunction of either PINK1 or Parkin likely results in the accumulation of low-quality mitochondria, thereby triggering early-onset familial PD. According to the most recently proposed model, selective localization of PINK1 to low-quality mitochondria facilitates the recruitment of cytosolic Parkin to the same mitochondria [6] , [7] , [8] , [9] , [10] , [11] , [12] . The ubiquitin ligase activity of Parkin, which is repressed under normal conditions, is re-established on damaged mitochondria [6] , [13] . Active Parkin then ubiquitylates mitochondrial outer membranous proteins such as Mitofusin, Miro and voltage-dependent anion channel [7] , [9] , [10] , [14] , [15] , [16] , [17] , [18] , [19] , [20] , [21] . The ubiquitylated proteins and damaged mitochondria are then degraded via the proteasome and autophagy, although the role of PINK1/Parkin in neurons remains controversial [5] , [19] , [22] , [23] , [24] , [25] . PD-associated PINK1 and Parkin mutations interfere with the ubiquitylation of depolarized mitochondria, suggesting the etiological importance of this process [6] , [7] , [8] , [9] , [12] . During this process, the principal initiation event is the discrimination of damaged mitochondria from their healthy counterparts. A model for this process has recently been described by Youle's group, in which newly synthesized PINK1 is imported to the inner membrane of healthy mitochondria and undergoes mitochondrial protease-dependent cleavage of its amino-terminal domain; the resulting truncated PINK1 is subsequently degraded by the proteasome [26] , [27] , [28] , [29] , [30] . However, because the ΔΨm is required for import, dissipation of ΔΨm prevents PINK1 from reaching the inner membrane. As a consequence, PINK1 remains localized to the outer mitochondrial membrane [31] , [32] , [33] . Although this model elegantly explains how the loss of ΔΨm causes the accumulation of PINK1 on damaged mitochondria, the molecular mechanisms underlying PINK1 retrieval of Parkin to depolarized mitochondria remain poorly understood. In this study, we identified two Ser residues (Ser228 and Ser402) in PINK1 that undergo autophosphorylation upon dissipation of mitochondrial ΔΨm in cells and determined that these autophosphorylation events are imperative for the efficient retrieval of Parkin to the same mitochondria. PINK1 regulation by mitochondrial ΔΨm If the essence of PINK1 regulation by mitochondrial ΔΨm is only the accumulation of PINK1, increasing the amount of PINK1 should bypass the requirement of ΔΨm to recruit Parkin onto mitochondria. When green fluorescent protein (GFP)-Parkin and PINK1 were co-transfected in HeLa cells under the control of a strong cytomegalovirus (CMV)-derived promoter, GFP-Parkin localized on mitochondria regardless of ΔΨm as reported previously [7] . However, the Parkin-recruitment activity of over-produced PINK1 was less than the Parkin-recruitment activity of endogenous PINK1 in the presence of the mitochondrial uncoupler carbonyl cyanide m -chlorophenylhydrazone (CCCP; Fig. 1a ), as immunoblotting confirmed that the amount of exogenous wild-type (WT) PINK1 was much more than that of endogenous PINK1 ( Fig. 1b , compare lane 1 with 3). This result indicates that endogenous PINK1 in the presence of the uncoupler more efficiently recruits Parkin to mitochondria than exogenous over-produced PINK1 in the absence of the uncoupler, and suggests that PINK1 is regulated not only quantitatively but also qualitatively in response to a decrease in mitochondrial ΔΨm. 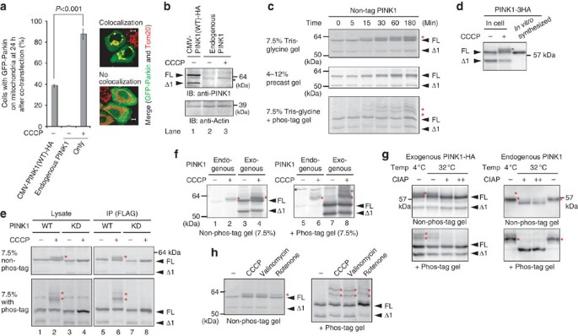Figure 1: PINK1 is phosphorylated following a decrease in mitochondrial ΔΨm. (a) Endogenous PINK1 in the presence of CCCP (10 μM, 1 h) recruits Parkin to mitochondria more efficiently than over-produced PINK1 (CMV promoter-driven) in the absence of CCCP. The number of cells with Parkin-positive mitochondria in the Parkin-expressing cells was counted in >100 cells. Error bars represent the mean±s.d. values of three experiments. Statistical significance was calculated using analysis of variance with a Tukey–Kramerpost hoctest. Example figures indicative of colocalization and no colocalization are shown on the right (scale bars, 10 μm). (b) Immunoblotting of exogenous and endogenous PINK1. The asterisk indicates the position of endogenous PINK1. Actin was used as a loading control. FL, full-length PINK1; Δ1, the N-terminal processed form. (c) HeLa cells expressing non-tagged PINK1 were treated with 10 μM CCCP for the indicated times and subjected to SDS–PAGE on a 7.5% Tris-glycine gel, a 4–12% precast gel or a 50 μM phos-tag containing gel. Red asterisks show phosphorylated PINK1. We routinely used HeLa cells and immunoblotting analysis was conducted with an anti-PINK1 antibody unless otherwise specified. (d)In vitrosynthesized PINK1-3HA and the mitochondrial fraction of PINK1-3HA-expressing cells following CCCP treatment were subjected to immunoblotting. (e) The cell lysate and immunoprecipitated product ofPINK1−/−MEFs-expressing WT or the PINK1 KD mutant were subjected to SDS–PAGE on a 7.5% Tris-glycine gel ±50 μM phos-tag. Red asterisks show phosphorylated PINK1. (f) The endogenous PINK1 in HeLa cells exists as the phosphorylated form. The black asterisk indicates a cross-reacting band and red asterisks show phosphorylated PINK1. (g) Phosphatase treatment caused the high-molecular shift of both exogenous and endogenous PINK1 to disappear. The mitochondrial fraction collected from HeLa cells-expressing PINK1-HA or collected from noninfected HeLa cells was treated with CIAP at the indicated temperature. Exogenous PINK1 was detected with an anti-HA antibody. + and ++ mean 10 and 30 U per reaction of CIAP, respectively. (h) Cells expressing exogenous PINK1 were treated with CCCP (10 μM, 1 h), valinomycin (10 μM, 1 h) or rotenone (200 μM, 24 h) and subjected to SDS–PAGE on a 7.5% Tris-glycine gel ±50 μM phos-tag. Figure 1: PINK1 is phosphorylated following a decrease in mitochondrial ΔΨm. ( a ) Endogenous PINK1 in the presence of CCCP (10 μM, 1 h) recruits Parkin to mitochondria more efficiently than over-produced PINK1 (CMV promoter-driven) in the absence of CCCP. The number of cells with Parkin-positive mitochondria in the Parkin-expressing cells was counted in >100 cells. Error bars represent the mean±s.d. values of three experiments. Statistical significance was calculated using analysis of variance with a Tukey–Kramer post hoc test. Example figures indicative of colocalization and no colocalization are shown on the right (scale bars, 10 μm). ( b ) Immunoblotting of exogenous and endogenous PINK1. The asterisk indicates the position of endogenous PINK1. Actin was used as a loading control. FL, full-length PINK1; Δ1, the N-terminal processed form. ( c ) HeLa cells expressing non-tagged PINK1 were treated with 10 μM CCCP for the indicated times and subjected to SDS–PAGE on a 7.5% Tris-glycine gel, a 4–12% precast gel or a 50 μM phos-tag containing gel. Red asterisks show phosphorylated PINK1. We routinely used HeLa cells and immunoblotting analysis was conducted with an anti-PINK1 antibody unless otherwise specified. ( d ) In vitro synthesized PINK1-3HA and the mitochondrial fraction of PINK1-3HA-expressing cells following CCCP treatment were subjected to immunoblotting. ( e ) The cell lysate and immunoprecipitated product of PINK1 −/− MEFs-expressing WT or the PINK1 KD mutant were subjected to SDS–PAGE on a 7.5% Tris-glycine gel ±50 μM phos-tag. Red asterisks show phosphorylated PINK1. ( f ) The endogenous PINK1 in HeLa cells exists as the phosphorylated form. The black asterisk indicates a cross-reacting band and red asterisks show phosphorylated PINK1. ( g ) Phosphatase treatment caused the high-molecular shift of both exogenous and endogenous PINK1 to disappear. The mitochondrial fraction collected from HeLa cells-expressing PINK1-HA or collected from noninfected HeLa cells was treated with CIAP at the indicated temperature. Exogenous PINK1 was detected with an anti-HA antibody. + and ++ mean 10 and 30 U per reaction of CIAP, respectively. ( h ) Cells expressing exogenous PINK1 were treated with CCCP (10 μM, 1 h), valinomycin (10 μM, 1 h) or rotenone (200 μM, 24 h) and subjected to SDS–PAGE on a 7.5% Tris-glycine gel ±50 μM phos-tag. Full size image We next examined how aside from quantitative regulation PINK1 is regulated by the mitochondrial ΔΨm. When HeLa cells harboring exogenous PINK1 were treated with CCCP, we realized that full-length PINK1 resolves as a doublet in immunoblots on conventional handmade 7.5% gels ( Fig. 1c ). The higher-molecular-weight band is rapidly observed within 30 min of CCCP treatment. This doublet is poorly resolved on commercially available precast gels ( Fig. 1c ), thus explaining why the doublet was not clear in our previous work [6] . Doublet formation of PINK1 is not derived from processing but rather results from post-translational modification because the molecular size of in vitro synthesized PINK1 corresponds to that of the lower PINK1 doublet band ( Fig. 1d ). To determine whether phosphorylation accounts for this modification, we performed electrophoresis using polyacrylamide gels conjugated with a 1,3-bis(bis(pyridin-2-ylmethyl)amino)propan-2-olato diMn(II) complex (referred to hereafter as Phos-tag). Phos-tag can capture phosphomonoester dianions (ROPO 3 2− ) and thus acrylamide-pendant phos-tag specifically retards the migration of phosphorylated proteins, which are visualized as slower-migrating bands compared with the corresponding nonphosphorylated proteins [34] . When exogenous PINK1 was subjected to polyacrylamide gel electrophoresis (PAGE)-containing phos-tag, a clear mobility shift of full-length PINK1 was observed, suggesting that PINK1 is phosphorylated following CCCP treatment (phos-tag panel of Fig. 1c , shown by red asterisks). PINK1 phosphorylation likely involves multiple sites because two higher-molecular-weight bands are observed. We next examined whether a kinase-dead (KD) mutation (K219A, D362A and D384A) that abolishes PINK1 kinase activity [35] prevents the appearance of this phosphorylated band. To avoid the effects of endogenous PINK1, we used mouse embryonic fibroblasts (MEFs) derived from a PINK1 knockout ( PINK1 −/− ) mouse [36] transformed with PINK1-Flag. In those cells, CCCP treatment resulted in a PINK1 doublet on a conventional 7.5% PAGE with the upper band clearly retarded in phos-tag-PAGE ( Fig. 1e , asterisks in lane 2). The phosphorylated PINK1 band, however, was completely absent on both 7.5% and phos-tag PAGE in the KD mutant ( Fig. 1e , lane 4), suggesting autophosphorylation. Clearer results were obtained following immunoprecipitation with an anti-Flag antibody ( Fig. 1e , lanes 5–8). We next checked whether endogenous PINK1 is also phosphorylated. As reported previously, the endogenous PINK1 signal was barely detectable under steady-state healthy conditions (lane 1 of Fig. 1f ), whereas CCCP treatment promoted the emergence of endogenous PINK1 (indicated by the red asterisk in lane 2 of Fig. 1f ) [6] , [7] , [37] , [38] . Compared with exogenous non-tagged PINK1, CCCP treatment caused endogenous PINK1 to resolve at a slightly higher-molecular weight (compare lane 2 with 3 of Fig. 1f ) and its mobility was consistent with the upper phosphorylated form of exogenous non-tagged PINK1 (compare lane 2 with 4). Phos-tag PAGE confirmed that the endogenous PINK1 that accumulated following CCCP treatment is the phosphorylated form ( Fig. 1f , lanes 6–8). To more convincingly demonstrate that PINK1 is phosphorylated, a mitochondrial fraction prepared from CCCP-treated cells was incubated with calf intestinal alkaline phosphatase (CIAP). This abolished the high-molecular-weight shift of not only exogenous PINK1 but also endogenous PINK1 ( Fig. 1g ). PINK1 phosphorylation was also observed when cells were treated with valinomycin (another type of mitochondrial uncoupler that functions as a K + uniporter) or rotenone (a mitochondrial complex I inhibitor), confirming that phosphorylation is not a CCCP-specific event ( Fig. 1h , red asterisks). Taken together, these results suggest that PINK1 undergoes autophosphorylation when the ΔΨm is decreased. PINK1 mutations can interfere with autophosphorylation To determine whether the aforementioned event is physiologically and pathologically significant, we examined the phosphorylation status of PINK1 harboring various pathogenic mutations that cause early-onset familial PD. We studied nine pathogenic missense mutations; that is, PINK1 harboring the C92F, A168P, E240K, H271Q, G309D, L347P, G386A, G409V or E417G mutations. We also used one pathogenic mutant with an amino-acid insertion in which a CAA codon (coding for glutamine) was inserted upstream of nucleotide 1602 (cytosine) and as a result glutamine was inserted within the carboxy-terminal domain at position 534 (referred to here after as 534insQ) [39] . These PINK1 mutants were serially introduced into HeLa cells, treated with CCCP and their phosphorylation status examined. PINK1 with the C92F mutation underwent phosphorylation in a manner equivalent to WT PINK1 ( Fig. 2a , lane 3). The band pattern of the G309D mutant was different from WT PINK1 in phos-tag PAGE, that is, slower-migrating bands (especially the upper band) were fainter in the G309D mutant than the WT PINK1 (phos-tag panel of Fig. 2a , lane 7). This result suggests that WT PINK1 is multiply phosphorylated whereas phosphorylation of the G309D mutant appears to be not as extensive. In the other pathogenic mutations, PINK1 phosphorylation was severely compromised ( Fig. 2a ) even though they localized on depolarized mitochondria ( Supplementary Fig. S1 ). Among the pathogenic mutations, the A168P, E240K, G386A and E417G mutations are expected to perturb the Mg 2+ /ATP-binding pocket of PINK1 [40] , again suggesting that phosphorylation of PINK1 is derived from autophosphorylation. We next checked the subcellular localization and autoubiquitylation of GFP-Parkin when the aforementioned PINK1 mutants were co-expressed in cells. We previously reported that the latent E3 activity of Parkin is activated upon recruitment to damaged mitochondria; as a consequence, autoubiquitylation of GFP-Parkin would be expected to be a good index of its mitochondrial localization [6] . In PINK1 −/− MEFs co-expressing the various PINK1 mutants, only the C92F mutant exhibited autoubiquitylation of GFP-Parkin equivalent to WT PINK1 ( Fig. 2b , lane 4). The G309D, E417G and 534insQ mutants showed weakened autoubiquitylation (lanes 8, 12 and 13). In contrast, the other PINK1 mutations severely hindered ubiquitylation of GFP-Parkin. Immunoblots confirmed that these mutants were expressed ( Fig. 2b ). Immunocytochemistry also confirmed the above results. Statistical analysis showed that co-expression of the C92F mutant resulted in the mitochondrial localization of GFP-Parkin, whereas the G309D, E417G and 534insQ mutants were unable to fully promote the mitochondrial localization of Parkin and the other pathogenic mutations failed to recruit GFP-Parkin to the mitochondria ( Fig. 2c ). These results showed that most pathogenic mutations compromised both the autophosphorylation activity of PINK1 and mitochondrial localization of Parkin. 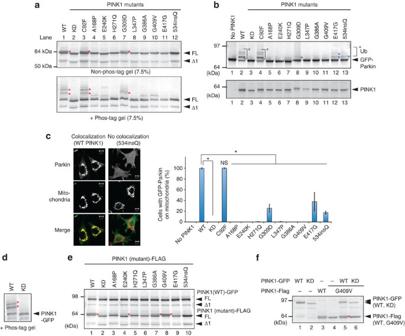Figure 2: PINK1 phosphorylation on damaged mitochondria is inhibited by most pathogenic mutations. (a) HeLa cells expressing PINK1-Flag with various pathogenic mutations were treated with CCCP, subjected to SDS–PAGE ± phos-tag and immunoblotted using an anti-PINK1 antibody. Red asterisks show phosphorylated PINK1. (b)PINK1−/−MEFs co-expressing GFP-Parkin and various pathogenic PINK1 mutants were subjected to non phos-tag PAGE and immunoblotting with anti-Parkin and anti-PINK1 antibodies. Blue asterisks show autoubiquitylation of GFP-Parkin, which is taken as evidence of its mitochondrial localization. (c) The subcellular localization of GFP-Parkin inPINK1−/−MEFs co-expressing various PINK1 mutants. Example figures indicative of colocalization and no colocalization are shown (bars, 10 μm). The number of cells with Parkin-positive mitochondria in the Parkin-expressing cells was counted in >100 cells. Error bars represent the mean±s.d. values of three experiments. Statistical significance was calculated using analysis of variance with a Tukey–Kramerpost hoctest; *P<0.01; ns, not significant. (d) PINK1-GFP undergoes auto-phosphorylation following CCCP treatment. Red asterisks show the phosphorylated PINK1-GFP. (e) Various pathogenic PINK1 mutants were co-transfected with PINK1(WT)-GFP, treated with CCCP and subjected to immunoblotting using an anti-PINK1 antibody. Red asterisks show the phosphorylated bands. (f) HeLa cells expressing PINK1(G409V)-Flag with PINK1-GFP or PINK1(KD)-GFP were treated with CCCP and subjected to conventional PAGE. Red asterisks show phosphorylated PINK1(G409V)-Flag. FL, Δ1 and KD represent full-length PINK1, N-terminal processed PINK1 and KD mutant, respectively. Figure 2: PINK1 phosphorylation on damaged mitochondria is inhibited by most pathogenic mutations. ( a ) HeLa cells expressing PINK1-Flag with various pathogenic mutations were treated with CCCP, subjected to SDS–PAGE ± phos-tag and immunoblotted using an anti-PINK1 antibody. Red asterisks show phosphorylated PINK1. ( b ) PINK1 −/− MEFs co-expressing GFP-Parkin and various pathogenic PINK1 mutants were subjected to non phos-tag PAGE and immunoblotting with anti-Parkin and anti-PINK1 antibodies. Blue asterisks show autoubiquitylation of GFP-Parkin, which is taken as evidence of its mitochondrial localization. ( c ) The subcellular localization of GFP-Parkin in PINK1 −/− MEFs co-expressing various PINK1 mutants. Example figures indicative of colocalization and no colocalization are shown (bars, 10 μm). The number of cells with Parkin-positive mitochondria in the Parkin-expressing cells was counted in >100 cells. Error bars represent the mean±s.d. values of three experiments. Statistical significance was calculated using analysis of variance with a Tukey–Kramer post hoc test; * P <0.01; ns, not significant. ( d ) PINK1-GFP undergoes auto-phosphorylation following CCCP treatment. Red asterisks show the phosphorylated PINK1-GFP. ( e ) Various pathogenic PINK1 mutants were co-transfected with PINK1(WT)-GFP, treated with CCCP and subjected to immunoblotting using an anti-PINK1 antibody. Red asterisks show the phosphorylated bands. ( f ) HeLa cells expressing PINK1(G409V)-Flag with PINK1-GFP or PINK1(KD)-GFP were treated with CCCP and subjected to conventional PAGE. Red asterisks show phosphorylated PINK1(G409V)-Flag. FL, Δ1 and KD represent full-length PINK1, N-terminal processed PINK1 and KD mutant, respectively. Full size image We next analysed the mode of PINK1 phosphorylation. As the activity of many kinases is regulated by intermolecular interactions [41] , we examined if the auto-phosphorylation of mutant PINK1 is ameliorated by co-expression with WT PINK1. When C-terminal GFP-tagged PINK1 (hereafter referred to as PINK1-GFP) was treated with CCCP and subjected to immunoblotting in the presence of phos-tag, slower-migrating phosphorylated bands were observed. These bands disappeared in the KD mutant, confirming that PINK1-GFP is functional and undergoes auto-phosphorylation ( Fig. 2d ). Next, PINK1-FLAG constructs harboring the various pathogenic mutations were transfected into HeLa cells with PINK1-GFP, treated with CCCP and then immunoblotted. As shown in Fig. 2e , while the majority of the mutants did not undergo phosphorylation in the presence of PINK1-GFP, a clear doublet was observed with the G409V PINK1 mutant (lane 8) and faint but reproducible doublet bands were also observed with the E240K and G386A mutants (lanes 4 and 7). Neither PINK1(G409V) alone nor co-expressed with PINK1(KD)-GFP underwent phosphorylation equivalent to WT PINK1 (lanes 4 and 6 of Fig. 2f ). In contrast, PINK1(G409V) was clearly phosphorylated when WT PINK1-GFP was co-expressed (lane 5). These results suggest that autophosphorylation can occur in trans between two PINK1 molecules. Ser228 and Ser402 are autophosphorylation sites of PINK1 We next sought to identify the PINK1 autophosphorylation site(s). As Ser/Thr residues in the activation loop of kinases are the most common and best-understood phosphorylation sites (for a review, see Huse and Kuriyan [42] and Nolen et al . [43] ), we decided to focus on the PINK1 activation loop. In the case of PINK1, the region spanning amino-acid residues 384–417 (384DFG ... APE417) corresponds to the activation loop. Three Ser residues (Ser393, Ser401 and Ser402) are present within this region. We consequently exchanged these Ser residues for Ala. PINK1 with either the S393A or the S401A mutation still underwent phosphorylation in a manner similar to WT PINK1 ( Fig. 3a , compare lanes 3 and 4 with lane 2). In contrast, the S402A mutation altered the band pattern of PINK1 (lane 5) with the upper band absent as assessed by conventional PAGE (non-phos-tag panel of Fig. 3a ). The S402A mutation likewise affected the banding pattern on the phos-tag PAGE gel (phos-tag panel of Fig. 3a ), with the emergence of a lower-molecular-weight band (black asterisk) slightly below the first band (red asterisk), which was absent in the mutation. Double and triple combinations of the S393A, S401A and S402A mutations failed to generate results that differed from the S402A mutation alone (lanes 7–9). The Ser residue at this position (402 in humans) is well conserved from mammals to nematodes, suggesting its physiological importance ( Fig. 3b ). The S402A mutation, however, did not impact all of the phosphorylation bands ( Fig. 3a ), suggesting that while S402 in the activation loop is dominantly phosphorylated, another PINK1 phosphorylation site is also utilized. 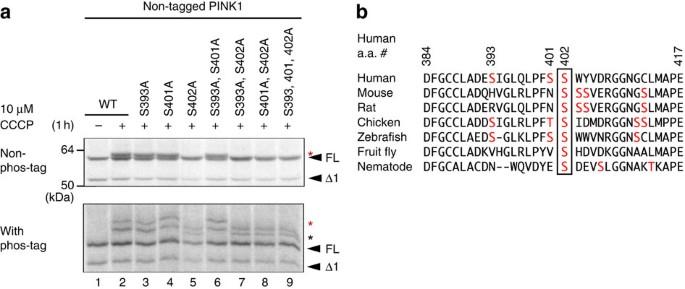Figure 3: S402A mutation partly inhibits the autophosphorylation of PINK1. (a) The S402A mutation altered the phosphorylation pattern of PINK1. PINK1 with the indicated mutations were transfected into HeLa cells and then subjected to SDS–PAGE on a 7.5% Tris-glycine gel ±50 μM phos-tag. Asterisks indicate phosphorylated PINK1 (see details of red and black asterisks in the text). (b) Ser/Thr residues in the activation loop of PINK1 from various organisms are shown in red font. Ser402 (boxed) is evolutionarily conserved. Figure 3: S402A mutation partly inhibits the autophosphorylation of PINK1. ( a ) The S402A mutation altered the phosphorylation pattern of PINK1. PINK1 with the indicated mutations were transfected into HeLa cells and then subjected to SDS–PAGE on a 7.5% Tris-glycine gel ±50 μM phos-tag. Asterisks indicate phosphorylated PINK1 (see details of red and black asterisks in the text). ( b ) Ser/Thr residues in the activation loop of PINK1 from various organisms are shown in red font. Ser402 (boxed) is evolutionarily conserved. Full size image To identify the other phosphorylation site, we performed mass spectrometric analysis of autophosphorylated PINK1. Glutathione S -transferase (GST)-fused PINK1 was integrated into the genome of HEK293 cells by retrovirus-mediated transformation. PINK1-GST was then purified from this stable cell line following +/− CCCP treatment ( Supplementary Fig. S2 ) and subjected to LC-MS/MS analysis after Asp-N protease digestion. A peptide equivalent to amino acids 206–230 (ERAPGAPAFPLAIKMMWNISAGSSS) was identified as a putative phosphorylated peptide. Although the unphosphorylated peptide was detected from both CCCP-treated and -untreated cells, the phosphorylated peptide was only detected from CCCP-treated cells ( Fig. 4a ). The MS/MS data suggested that Ser228, Ser229 or Ser230 was phosphorylated; more specific determination of the phosphorylation site is problematic ( Fig. 4b ). These candidate Ser residues have been relatively conserved during evolution ( Fig. 4c ). A peptide containing phospho-Ser402 was not identified in this analysis, possibly because the signal intensity was below the threshold of detection. 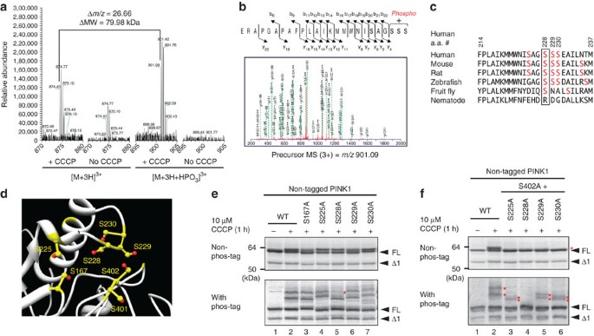Figure 4: S228 is another autophosphorylation site for PINK1. (a) Mass spectrometric analysis of thein vivoautophosphorylation site of PINK1. PINK1-GST purified from cells +/−CCCP treatment was subjected to LC-MS/MS analysis with a phosphorylated peptide equivalent to amino acids 206–230 detected only from CCCP-treated cells. (b) The MS/MS data suggested that phosphorylation occurs at Ser228, Ser229 or Ser230. (c) Multiple sequence alignment of PINK1 residues neighboring Ser228 from various organisms. Ser228 (boxed) has been evolutionarily conserved across most species. (d) Structural model (Protein Model Database ID: PM0076345) of PINK1 revealed that the possible phosphorylation sites including S228 and S402 are spatially close to one another. Ser residues are shown in yellow and hydroxyl groups are highlighted in red. (e) The S228A mutation changed the phosphorylation pattern of PINK1. The first band (shown by a red asterisk) in phos-tag PAGE is not observed in cell expressing the S228A mutation. (f) Autophosphorylation-derived signals of PINK1 in cells expressing the S228A/S402A double mutation are completely abolished. Asterisks indicate the phosphorylated form. Figure 4: S228 is another autophosphorylation site for PINK1. ( a ) Mass spectrometric analysis of the in vivo autophosphorylation site of PINK1. PINK1-GST purified from cells +/−CCCP treatment was subjected to LC-MS/MS analysis with a phosphorylated peptide equivalent to amino acids 206–230 detected only from CCCP-treated cells. ( b ) The MS/MS data suggested that phosphorylation occurs at Ser228, Ser229 or Ser230. ( c ) Multiple sequence alignment of PINK1 residues neighboring Ser228 from various organisms. Ser228 (boxed) has been evolutionarily conserved across most species. ( d ) Structural model (Protein Model Database ID: PM0076345) of PINK1 revealed that the possible phosphorylation sites including S228 and S402 are spatially close to one another. Ser residues are shown in yellow and hydroxyl groups are highlighted in red. ( e ) The S228A mutation changed the phosphorylation pattern of PINK1. The first band (shown by a red asterisk) in phos-tag PAGE is not observed in cell expressing the S228A mutation. ( f ) Autophosphorylation-derived signals of PINK1 in cells expressing the S228A/S402A double mutation are completely abolished. Asterisks indicate the phosphorylated form. Full size image Although the three-dimensional structure of PINK1 has not yet been solved, a reliable structural model based on the structure of a related kinase (CaMKII) has been deposited in the Protein Model Database (accession code: PM0076345) [44] . Unexpectedly, we found that Ser228, Ser229 and Ser230 localized very close to Ser402 ( Fig. 4d ) and that they constituted a small structural patch on the surface of the PINK1 model ( Supplementary Fig. S3 ). These Ser residues, as well as the spatially close Ser167 and Ser225, were serially exchanged for Ala. PINK1 with the S167A, S225A, S229A or S230A mutation showed double phosphorylated bands in phos-tag PAGE, although the molecular weight of those bands was altered to some degree ( Fig. 4e ). In contrast, the first band in phos-tag PAGE (red asterisk in Fig. 4e ) disappeared in the S228A mutation (note that a faint band near the asterisk is a cross-reacting band also observed in lane 1 (WT)). Moreover, the PINK1 autophosphorylation signal was completely absent in the S228A/S402A double mutant ( Fig. 4f , lane 4). Combining the S225A, S229A and S230A mutations with the S402A mutation had no such effect on the autophosphorylation signal ( Fig. 4f , lanes 3, 5 and 6) and were almost indistinguishable from the S402A mutation alone ( Fig. 3a , lanes 5). These results indicate that S228 and S402 are PINK1 autophosphorylation sites. PINK1 autophosphorylation recruits Parkin to the mitochondria Next, we sought to determine whether autophosphorylation of PINK1 is important to recruit Parkin to mitochondria. However, this experiment presents a unique challenge in that overexpression of exogenous PINK1 itself results in the targeting of Parkin to mitochondria irrespective of the mitochondrial ΔΨm [7] , [45] , [46] and autophosphorylation ( Fig. 1 ). We thus attempted to establish an experimental system in which Parkin does not migrate to the healthy mitochondria even in the presence of exogenously expressed PINK1. When WT PINK1 was expressed under a strong CMV promoter, a significant amount of co-transfected GFP-Parkin was recruited to the mitochondria even without CCCP treatment ( Fig. 5a , the second bar). Therefore, we modified the CMV promoter to reduce expression and found that deletion of the enhancer region in the plasmid (referred to as CMV(d1) hereafter) significantly attenuated PINK1 expression (anti-PINK1 panel of Fig. 5b , compare lane 2 with 3). With this attenuated CMV(d1) promoter, at 24 h post transfection, we observed almost no recruitment of co-expressed GFP-Parkin to mitochondria by the WT PINK1 ( Fig. 5a , the third bar). We also checked the autoubiquitylation status of GFP-Parkin, a good index of its mitochondrial localization [6] , and confirmed that GFP-Parkin exhibits autoubiquitylation when co-expressed with PINK1 under the control of a CMV promoter, whereas the autoubiquitylation was hardly observed with PINK1 under the control of the CMV(d1) promoter (anti-Parkin panel of Fig. 5b ). Moreover, when PINK1 −/− MEFs co-expressing GFP-Parkin and CMV(d1) promoter-driven PINK1 were treated with CCCP, autoubiquitylation of GFP-Parkin was clearly observed only following CCCP treatment ( Fig. 5c , lane 4), suggesting that a defined expression level of exogenous PINK1 enables Parkin to localize specifically to depolarized mitochondria. 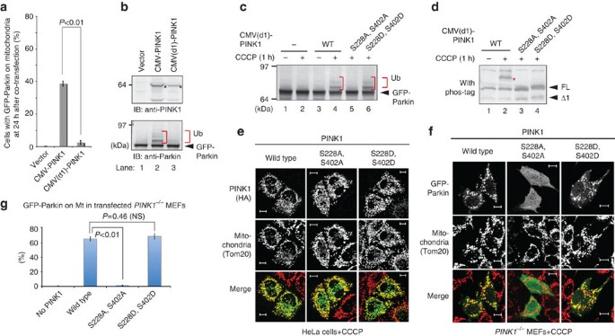Figure 5: PINK1 autophosphorylation of S228/S402 is essential for mitochondrial localization of Parkin. (a) HeLa cells were co-transfected with GFP-Parkin and CMV or CMV(d1) promoter-driven PINK1. The number of cells with Parkin-positive mitochondria was counted in >100 cells at 24 h post transfection. Error bars represent the mean±s.d. values of three experiments. Statistical significance was calculated using analysis of variance with a Tukey–Kramerpost hoctest. (b) Immunoblotting with an anti-PINK1 antibody to measure the quantity of PINK1 (marked by asterisks) expressed by the CMV or CMV(d1) promoter, and autoubiquitylation activity of GFP-Parkin when the indicated PINK1 plasmids were co-transfected. The slower-migrating bands were derived from ubiquitylation (Ub). (c)PINK1−/−MEFs co-expressing GFP-Parkin and CMV(d1) promoter-driven PINK1 harboring the S228A/S402A or S228D/S402D mutation were subjected to immunoblotting with an anti-Parkin antibody. Ub shows autoubiquitylation of GFP-Parkin, which is taken as an indicator of its mitochondrial localization. (d) Both the S228A/S402A and S228D/S402D mutations hindered autophosphorylation of PINK1 in phos-tag PAGE. The asterisk indicates the phosphorylated form. FL and Δ1 mean full-length and N-terminal processed PINK1, respectively. (e) Subcellular localization of indicated PINK1 mutants in HeLa cells following CCCP treatment. Immunocytochemistry confirmed that both of the S228A/S402A and S228D/S402D PINK1 mutants localized on mitochondria following CCCP treatment. Bars, 10 μm. (f) Subcellular localization of GFP-Parkin inPINK1−/−MEFs co-expressing CMV(d1) promoter-driven PINK1 harboring the S228A/S402A or S228D/S402D mutation. Immunocytochemistry showing that the S228A/S402A PINK1 mutant disturbed the mitochondrial localization of Parkin, whereas the S228D/S402D mutant recruited Parkin to the mitochondria equivalent to WT PINK1. Bars, 10 μm. (g) The number of cells with Parkin-positive mitochondria was counted in >100 cells following CCCP treatment. Statistical analysis was performed as in (a). Figure 5: PINK1 autophosphorylation of S228/S402 is essential for mitochondrial localization of Parkin. ( a ) HeLa cells were co-transfected with GFP-Parkin and CMV or CMV(d1) promoter-driven PINK1. The number of cells with Parkin-positive mitochondria was counted in >100 cells at 24 h post transfection. Error bars represent the mean±s.d. values of three experiments. Statistical significance was calculated using analysis of variance with a Tukey–Kramer post hoc test. ( b ) Immunoblotting with an anti-PINK1 antibody to measure the quantity of PINK1 (marked by asterisks) expressed by the CMV or CMV(d1) promoter, and autoubiquitylation activity of GFP-Parkin when the indicated PINK1 plasmids were co-transfected. The slower-migrating bands were derived from ubiquitylation (Ub). ( c ) PINK1 −/− MEFs co-expressing GFP-Parkin and CMV(d1) promoter-driven PINK1 harboring the S228A/S402A or S228D/S402D mutation were subjected to immunoblotting with an anti-Parkin antibody. Ub shows autoubiquitylation of GFP-Parkin, which is taken as an indicator of its mitochondrial localization. ( d ) Both the S228A/S402A and S228D/S402D mutations hindered autophosphorylation of PINK1 in phos-tag PAGE. The asterisk indicates the phosphorylated form. FL and Δ1 mean full-length and N-terminal processed PINK1, respectively. ( e ) Subcellular localization of indicated PINK1 mutants in HeLa cells following CCCP treatment. Immunocytochemistry confirmed that both of the S228A/S402A and S228D/S402D PINK1 mutants localized on mitochondria following CCCP treatment. Bars, 10 μm. ( f ) Subcellular localization of GFP-Parkin in PINK1 −/− MEFs co-expressing CMV(d1) promoter-driven PINK1 harboring the S228A/S402A or S228D/S402D mutation. Immunocytochemistry showing that the S228A/S402A PINK1 mutant disturbed the mitochondrial localization of Parkin, whereas the S228D/S402D mutant recruited Parkin to the mitochondria equivalent to WT PINK1. Bars, 10 μm. ( g ) The number of cells with Parkin-positive mitochondria was counted in >100 cells following CCCP treatment. Statistical analysis was performed as in ( a ). Full size image We next determined the effect of phosphorylation-deficient (Serine-to-Alanine) mutations or phosphorylation-mimic (Serine-to-Aspartic acid) mutations of Ser228 and Ser402 on Parkin recruitment. When PINK1 with either the S228A/S402A or the S228D/S402D double mutation was subjected to phos-tag PAGE, the autophosphorylation-derived PINK1 bands disappeared in both cases because the phosphorylation sites were missing ( Fig. 5d ). We then examined the Parkin-recruitment activity of these mutants. Importantly, the S228A/S402A mutant was unable to restore autoubiquitylation of GFP-Parkin in PINK1 −/− MEFs ( Fig. 5c , lane 5), whereas the S228D/S402D mutant complemented it ( Fig. 5c , lane 6), although neither underwent autophosphorylation ( Fig. 5d ). We confirmed that the PINK1 S228A/S402A mutant localized on mitochondria following CCCP treatment as well as WT PINK1 ( Fig. 5e ). Immunocytochemistry of Parkin further demonstrated that the PINK1 S228D/S402D mutant promoted mitochondrial localization of Parkin equivalent to WT PINK1, whereas the PINK1 S228A/S402A mutant failed to recruit Parkin onto mitochondria ( Fig. 5f,g ). The results shown in Fig. 5 reveal that autophosphorylation of PINK1 is indeed important for recruiting Parkin onto damaged mitochondria, and is the first evidence that autophosphorylation of PINK1 has a crucial role in the PINK1/Parkin pathway. Recently, our understanding of how PINK1 and Parkin function has undergone a significant transformation that continues to evolve. We can accurately state that PINK1 and Parkin function in maintaining mitochondrial integrity by cooperatively working together to identify and label damaged mitochondria via ubiquitylation (reviewed by refs 3 , 31 , 32 , 33 , 47 ). Biochemically, Parkin functions as an E3 enzyme that catalyses the transfer of ubiquitin from E1/E2~ubiquitin to the substrate [48] , [49] , whereas PINK1 is thought to possess Ser/Thr kinase activity. Although we and other investigators demonstrated that PINK1 is essential for the recruitment of Parkin to damaged mitochondria, the role of PINK1 kinase activity in Parkin recruitment remains to be fully addressed. Indeed, measurements of PINK1 kinase activity have been difficult and thus biochemical-based studies, especially in vivo , have not advanced enough. In this study, we addressed these problems and revealed several new findings. The solubilization and purification of full-length PINK1 has been difficult and thus almost all studies, excluding one exception [50] , of in vitro kinase activity have been done using a truncated PINK1 kinase domain [35] , [45] , [51] , [52] , [53] . Moreover, although several candidates have been reported [20] , [54] , the physiological substrate(s) of PINK1 in vivo remains controversial; as a consequence the role of PINK1 kinase activity has not been fully elucidated. In this study, we indicated that, once localized to depolarized mitochondria, PINK1 catalyses the intermolecular autophosphorylation of itself ( Figs 1 and 2 ), although other modes of phosphorylation by another kinases cannot be ruled out completely. To study the significance of this autophosphorylation, we sought to identify the autophosphorylation site(s). Mutational analyses indicated that Ser228 and Ser402 are the PINK1 autophosphorylation sites. Moreover, direct evidence for in vivo phosphorylation by mass spectrometric analysis was obtained for Ser228 ( Fig. 4 ). Although Muqit's lab [50] recently reported that insect ( Tribolium castaneum ) PINK1 catalysed autophosphorylation of Ser205 (equivalent to Ser228 in human PINK1) in vitro , our work provides the first direct evidence of autophosphorylation at Ser228 of PINK1 in vivo . Unfortunately, a peptide containing phospho-Ser402 was not identified in the MS analysis and thus the data are not as explicit as those of Ser228. However, mutational analyses suggest that both Ser228 and Ser402 are PINK1 phosphorylation sites ( Figs 3a , 4e and 4f ). Moreover, the PINK1 structural model predicts that these Ser residues are spatially very close and comprise a small patch on the surface, supporting the above conclusion ( Fig. 4d and Supplementary Fig. S3 ). It has been reported that when WT PINK1 or PINK1 continuously localized to mitochondria (OPA3-PINK1 chimera) is overexpressed in cells, Parkin localizes on the mitochondria irrespective of ΔΨm [7] , [45] , [46] . On the other hand, autophosphorylation was not induced by over-production ( Fig. 1 ), but did require a decrease in ΔΨm. This result seemingly suggests that autophosphorylation of PINK1 is not important for Parkin recruitment to mitochondria. However, we propose that autophosphorylation is indeed significant for three reasons. First, based on the phosphorylation status shown in Fig. 1f,g , almost all of the endogenous PINK1 is phosphorylated in a loss of ΔΨm-directed manner. Moreover, a majority of the pathogenic mutations severely compromised PINK1 autophosphorylation ( Fig. 2a ). Second, when the expression of exogenous PINK1 was under the control of the CMV(d1) promoter, Parkin mitochondrial localization coincided with PINK1 autophosphorylation ( Fig. 5c,d ). Third, a phosphorylation-deficient mutation of PINK1 (S228A/S402A) hindered the mitochondrial localization of Parkin, whereas a phosphorylation-mimic mutation of PINK1 (S228D/S402D) bypassed the necessity of PINK1 autophosphorylation for Parkin recruitment ( Fig. 5c–g ). Although the need for PINK1 autophosphorylation in recruiting Parkin can be suppressed by excessive over-production, we propose that PINK1 autophosphorylation under conditions such as dissipation of ΔΨm in the presence of endogenous PINK1, or the controlled, appropriate expression of exogenous PINK1 is more physiologically relevant. In the case of the MAP kinase extracellular signal-regulated kinase 2, its phosphorylation increases the k cat by ~1,000-fold relative to the unphosphorylated form [43] . Although the physiological relevance of PINK1 autophosphorylation is unknown, we speculate that the phosphorylation of PINK1 increases the k cat similar to extracellular signal-regulated kinase 2. This model is compatible with our observation described above that over-production of PINK1 suppresses the requirement of its phosphorylation. As described in the Introduction, the basic mechanisms connecting mitochondrial damage to PINK1 accumulation have recently been elucidated [31] . The essence of the prevailing model is that PINK1 monitors mitochondrial damage via its escape from ΔΨm-dependent import and degradation; namely, that dissipation of ΔΨm prevents PINK1 from reaching the inner membrane, and as a consequence PINK1 remains localized to the outer mitochondrial membrane and tethered to the TOM complex [55] . However, herein we have experimentally demonstrated that while the above monitoring route is necessary for the discrimination of damaged mitochondria it might not be sufficient for fulfilling downstream events such as Parkin recruitment to mitochondria. Indeed, the low-level (but more than endogenous-level) accumulation of nonphosphorylated PINK1 on the outer membrane (for example, CMV(d1) promoter-driven PINK1(S228A/S402A) following CCCP treatment) cannot retrieve cytosolic Parkin efficiently, and autophosphorylation of PINK1 (for example, CMV(d1) promoter-driven PINK1(S228D/S402D) or endogenous PINK1 following CCCP treatment) is an essential step for optimized Parkin recruitment. We propose that the integrity of the mitochondria is sensed by the escape from ΔΨm-dependent degradation and is transduced to Parkin via autophosphorylation of PINK1, as depicted in Fig. 6 . 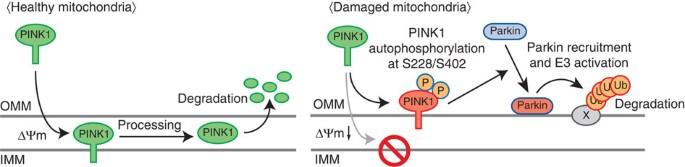Figure 6: A model for Parkin recruitment to the damaged mitochondria. The integrity of the mitochondria is sensed and transduced to Parkin by two sequential processes, that is the escape from membrane potential-dependent degradation and autophosphorylation of PINK1 at Ser228/Ser402. Both steps are essential for optimized Parkin recruitment and activation. Figure 6: A model for Parkin recruitment to the damaged mitochondria. The integrity of the mitochondria is sensed and transduced to Parkin by two sequential processes, that is the escape from membrane potential-dependent degradation and autophosphorylation of PINK1 at Ser228/Ser402. Both steps are essential for optimized Parkin recruitment and activation. Full size image Plasmids Plasmids used in this study are summarized in Supplementary Table S1 . To generate the plasmid for weak PINK1 expression, the Bgl II– Hin dIII fragment within the CMV promoter was excised from pCMVTNT (Promega) and refilled with a 130-bp DNA fragment amplified using the following primers: 5′-TTGTTAGATCTCCAAAATCAACGGGACTTTCCAA-3′ and 5′-AGTGCCTCACGACCAACTTCTG-3′ and digested with Bgl II and Hin dIII. As a result, the upstream 620 bp of the CMV promoter was deleted from pCMVTNT and the resulting plasmid was named pCMV(d1)TNT. Cells Various stable MEF transformants were established by infecting MEFs with recombinant retroviruses [6] , [56] . PINK1 and/or Parkin were cloned into a pMXs-puro vector. Retrovirus packaging cells PLAT-E [56] were transfected with the above vectors and were cultured at 37 °C for 24 h. After changing the medium, cells were further incubated at 37 °C for 24 h and the viral supernatant was collected and used for infection. MEFs were plated on 35-mm dishes at 24 h before infection, and the medium was replaced with the undiluted viral supernatant described above and 8 μg ml −1 polybrene (Sigma). After 2 days, transformants were selected in medium containing 5 μg ml −1 puromycin. HeLa cells stably expressing GFP-Parkin were established using recombinant retroviruses as well; however, as murine ecotropic retrovirus made by PLAT-E cells cannot infect HeLa cells, the retroviral receptor mCAT1 was transiently expressed in HeLa cells before viral infection. Plasmid transfection into HeLa cells and MEFs was performed using Fugene6 (Roche) and polyethylenimine (Polyscience), respectively. To depolarize the mitochondria, HeLa cells and MEFs were treated with 10 and 30 μM CCCP for 1–3 h. Phos-tag assay and CIAP treatment To detect phosphorylated proteins via PAGE, 7.5% polyacrylamide gels containing 50 μM phos-tag acrylamide (Wako chemicals) and 100 μM MnCl 2 were used. After electrophoresis, phos-tag acrylamide gels were washed with transfer buffer containing 0.01% SDS and 1 mM EDTA for 10 min with gentle shaking, and then replaced with transfer buffer containing 0.01% SDS without EDTA for 10 min according to the manufacturer's protocol. Proteins were transferred to polyvinylidene difluoride membranes and analysed by conventional immunoblotting. For CIAP treatment, a mitochondria-rich fraction (10 μg) collected by low-speed centrifugation from un-transfected or PINK1-3HA-transfected HeLa cells with CCCP treatment was incubated with 0, 10 or 30 U per reaction CIAP (Takara) for 1 h at the indicated temperature in reaction buffer (50 mM Tris–HCl pH 9.0, 1 mM MgCl 2 , and 0.3 M trehalose), and then subjected to standard PAGE or phos-tag PAGE containing 25 μM phos-tag acrylamide (Wako Chemicals) and 50 μM MnCl 2 and then immunoblotted. Immunofluorescence and immunoblotting To detect the autoubiquitylation of GFP-Parkin by immunoblotting (IB), the cell lysate of HeLa cells or MEFs was collected in the presence of 10 mM N -ethylmaleimide to protect ubiquitylated Parkin from deubiquitylation. For immunofluorescence (IF) experiments, cells were fixed with 4% paraformaldehyde, permeabilized with 50 μg ml −1 digitonin and stained with the primary antibodies described below and the following secondary antibodies: mouse and/or rabbit Alexa Fluor 488, 568 and 647 (Invitrogen, 1:2,000 dilution). Cells were imaged using a laser-scanning microscope (LSM510; Carl Zeiss, Inc.). Image contrast and brightness were adjusted in Photoshop (Adobe). Antibodies used are as follows: anti-FLAG (M2 agarose; Sigma, 1:80 dilution) for immunoprecipitation, anti-actin (AC-40; Sigma, 1:1,000 dilution), anti-HA (4B2; Wako chemicals, 1:250 dilution), anti-Parkin (PRK8; Sigma-Aldrich, 1:1,500 dilution) and anti-PINK1 (BC100-494; Novus, 1:1,000 dilution) for IB, anti-GFP (3E6; Wako chemicals, 1:1,000 dilution), anti-PINK1 (BC100-494; Novus, 1:200 dilution and N4/15; NeuroMab, 1:200 dilution) and anti-Tom20 (FL-145, 1:3,000 dilution and F-10, 1:200 dilution; Santa Cruz Biotechnology) for IF. Statistical comparisons were made using analysis of variance with a Tukey–Kramer post hoc test in the JMP8.0.1 software (SAS Institute Inc.). LC-MS/MS analysis of PINK1-GST PINK1-GST from CCCP-treated and -untreated cells was subjected to SDS–PAGE and stained with CBB. PINK1-GST protein bands were excised, reduced, alkylated and digested with endoproteinase Asp-N (Roche) in 12.5 mM ammonium bicarbonate, pH 8.0, and 5 mM Tris–Cl for 16 h at 37 °C. The resultant peptides were analysed on an LTQ Orbitrap XL mass spectrometer (Thermo Scientific) with the raw data processed using Xcalibur (Thermo Scientific). The peak list files were searched against the NCBI nonredundant protein database restricted to Homo sapiens using the MS/MS ion search function of the Mascot search engine (Matrix Science). The 'Asp-N_ambic' enzyme parameter setting was selected for cleavage of peptide bonds N-terminally at both Asp and Glu residues. How to cite this article: Okatsu, K. et al . PINK1 autophosphorylation upon membrane potential dissipation is essential for Parkin recruitment to damaged mitochondria. Nat. Commun. 3:1016 doi: 10.1038/ncomms2016 (2012).